RSPO2–LGR5 signaling has tumour-suppressive activity in colorectal cancer R-spondins are a family of secreted Wnt agonists. One of the family members, R-spondin 2 (RSPO2), has an important role in embryonic development, bone formation and myogenic differentiation; however, its role in human cancers remains largely unknown. Here we show that RSPO2 expression is downregulated in human colorectal cancers (CRCs) due to promoter hypermethylation, and that the RSPO2 reduction correlates with tumour differentiation, size and metastasis. Overexpression of RSPO2 suppresses CRC cell proliferation and tumorigenicity, whereas the depletion of RSPO2 enhances tumour cell growth. RSPO2 has an inhibitory effect on Wnt/β-catenin signaling in the CRC cells that show suppressed cell proliferation. In human CRC cells, the RSPO2-induced inhibition of Wnt signaling depends on leucine-rich repeat-containing G-protein-coupled receptor 5 (LGR5); RSPO2 interacts with LGR5 to stabilize the membrane-associated zinc and ring finger 3 (ZNRF3). Our data suggest that RSPO2 functions as a tumour suppressor in human CRCs, and these data reveal a RSPO2-induced, LGR5-dependent Wnt signaling-negative feedback loop that exerts a net growth-suppressive effect on CRC cells. Colorectal cancer (CRC) is the third most common cancer worldwide [1] . A number of key oncogenes, tumour suppressor genes and pathways have been implicated in driving the transition from healthy colonic epithelium to malignant tumours; the Wnt pathway and its components have proven to be the most important [2] . Activation of the canonical Wnt/β-catenin pathway involves the interaction of Wnt ligands with cell-surface Frizzled receptors and LRP5/6 co-receptors. This interaction disrupts the APC/Axin/CK1a/GSK3β complex, thus resulting in the accumulation and translocation of β-catenin into the nucleus, where it activates target gene expression by interacting with TCF/LEF transcription factors [3] . The Wnt/β-catenin pathway plays a pivotal role in CRC tumorigenesis, and aberrant activation of the Wnt pathway is associated with ~90% of human CRCs [4] , [5] . R-spondins are a family of Wnt activators. The R-spondin family consists of four secreted proteins (RSPO1–4) that share 60% overall sequence homology and contain two furin-like cysteine-rich domains [6] , [7] . They were first discovered as Wnt agonists owing to their strong potentiation of canonical Wnt/β-catenin signaling [8] , [9] . Recently, R-spondins were identified as bona fide ligands of the leucine-rich repeat-containing G-protein-coupled receptors (LGRs), including LGR4, 5 and 6 (refs 10 , 11 , 12 ). Studies have characterized the role of R-spondins in various cellular and biological processes, such as sex determination [13] , cell proliferation [14] , embryonic development [15] , bone formation [16] , [17] , myogenic differentiation [18] and tumorigenesis [13] , [19] . Polymorphism in one of the R-spondin family members, RSPO2, leads to genetic susceptibility to Dupuytren’s disease in humans [20] . RSPO2 is also essential for vertebrate embryo development [21] , [22] , [23] . RSPO2 gene knockout mice die immediately after birth and display multiple abnormalities, including limb defects, craniofacial and laryngeal tracheal malformation and lung hypoplasia [22] , [24] , [25] . Over the last several years, research on RSPO2 has accumulated, especially with respect to its role in Wnt signaling activation. However, the role of RSPO2 in cancers remains poorly understood. RSPO2 was identified as a common integration site for mouse mammary tumours [26] , [27] . In a transposon-based genetic screen in mice, the RSPO2 gene was identified as the second best candidate CRC driver gene after Apc [28] . Furthermore, recurrent RSPO2 gene fusion occurs in colon tumours [29] . Together, these findings suggest that RSPO2 may play an important role in human CRC tumorigenesis. In this study, we investigated the functions of RSPO2 in human CRCs. We found that RSPO2 expression is downregulated in the majority of human CRCs due to promoter methylation. RSPO2 has an anti-oncogenic role in CRC tumour growth, depending on the presence of LGR5. In CRC cells that are competent for LGR5 expression, RSPO2 may function as a tumour suppressor by negatively regulating Wnt/β-catenin signaling through an LGR5-dependent feedback mechanism. RSPO2 is downregulated in human CRC cells and primary tumours Using RNAseq to investigate transcriptional regulation in CRC, we found that RSPO2 gene transcripts could not be detected in DLD1 cells (NCBI/SRA, accession number SRR1045067 ). RSPO2 is expressed in the gastrointestinal tract [30] ; in the normal intestine, RSPO2 is expressed in the crypt epithelial cells ( Supplementary Fig. 1 ). Thus, we sought to determine whether the downregulation or silencing of RSPO2 expression is a general feature of CRC cells, including those cells isolated from primary CRCs. Indeed, an initial survey of nine CRC cell lines revealed that, while RSPO2 could be readily detected in samples from normal colonic mucosa, its expression was significantly lower or undetectable in all nine CRC cell lines examined ( Fig. 1a ). Similarly, we found that in 68 of 80 (85%) primary CRC tumours, RSPO2 transcripts and proteins were both significantly downregulated in the tumour samples compared with their matched adjacent normal mucosa ( Fig. 1b–d ). 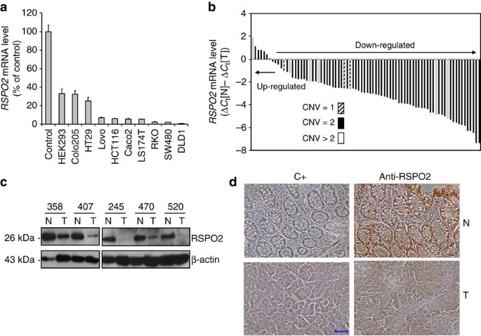Figure 1:RSPO2 expression is downregulated in CRC tumours. (a) Relative RSPO2 mRNA expression in CRC cell lines. RSPO2 mRNA levels were determined using qRT–PCR. Normal mucosa samples were used as a control (100%). Mean±s.d., data were calculated from triplicates. (b) qRT–PCR analysis of the relative RSPO2 mRNA expression in primary CRC tumours. The expression of RSPO2 was normalized to β-actin. Data were calculated from triplicates. Each bar represents the value of ΔΔCt=ΔCt[N]−ΔCt[T]. [T] represents colorectal tumour, and [N] is the matched normal mucosa. The copy number variation (CNV) of RSPO2 within the concomitant tumour genome was determined with TaqMan copy number assay. (c) Western blotting for RSPO2 protein in CRC tumours. The results from five randomly selected pairs of CRC tumours (T) and matched adjacent colonic mucosa (N) are presented. (d) Immunohistochemical staining of RSPO2 in CRC tumours (T) and matched normal mucosa (N). The C+ panel is the negative control without the anti-RSPO2 antibody. Scale bar: 50 μm. In addition, the statistical analysis revealed a significant association between the decreased expression of RSPO2 and tumour differentiation ( P <0.001), infiltration ( P <0.01), lymph node metastasis ( P <0.001) and tumour size ( P <0.001) ( χ 2 test) ( Table 1 ). Figure 1: RSPO2 expression is downregulated in CRC tumours . ( a ) Relative RSPO2 mRNA expression in CRC cell lines. RSPO2 mRNA levels were determined using qRT–PCR. Normal mucosa samples were used as a control (100%). Mean±s.d., data were calculated from triplicates. ( b ) qRT–PCR analysis of the relative RSPO2 mRNA expression in primary CRC tumours. The expression of RSPO2 was normalized to β-actin. Data were calculated from triplicates. Each bar represents the value of ΔΔ C t =Δ C t [N]−Δ C t [T]. [T] represents colorectal tumour, and [N] is the matched normal mucosa. The copy number variation (CNV) of RSPO2 within the concomitant tumour genome was determined with TaqMan copy number assay. ( c ) Western blotting for RSPO2 protein in CRC tumours. The results from five randomly selected pairs of CRC tumours (T) and matched adjacent colonic mucosa (N) are presented. ( d ) Immunohistochemical staining of RSPO2 in CRC tumours (T) and matched normal mucosa (N). The C+ panel is the negative control without the anti-RSPO2 antibody. Scale bar: 50 μm. Full size image Table 1 Relationship between expression levels of RSPO2 in CRC tumours and clinical and pathologic features of the individuals. Full size table Loss of RSPO2 is frequently due to promoter hypermethylation With the TaqMan copy number variation assay, we found no significant correlation between the copy number and mRNA levels of RSPO2 in 80 pairs of CRC tumour samples (Spearman P =0.922) ( Fig. 1b ). Resequencing of the cDNA and 5′ promoter region of RSPO2 also identified no genetic mutation that could result in RSPO2 silencing. These data are consistent with a previous study of 70 pairs of colon tumours by next-generation sequencing [29] . In human CRCs, a number of tumour suppressor genes are downregulated due to promoter methylation [31] . A careful examination of the RSPO2 promoter revealed that it contains a CpG island ( Fig. 2a ). Thus, we asked whether RSPO2 is targeted for methylation-mediated silencing. We found that treatment with 5-Aza-dC restored RSPO2 expression in both LS174T and DLD1 cells ( Fig. 2b ). Moreover, bisulphite sequencing confirmed that the CpG islands of the RSPO2 promoter in CRC cells were hypermethylated ( Fig. 2c ). We then developed a methylation-specific PCR (MSP) assay and surveyed RSPO2 promoter methylation in additional CRC cell lines and primary tissue samples. We found that MSP-specific products were detected in all nine CRC cell lines examined and in 61 of 80 (76%) primary tumour samples ( Fig. 2d ). The bisulphite sequencing analysis of three normal mucosa-CRC tumour pairs confirmed the presence of extensive methylation in the tumour samples but infrequent methylation in the matched mucosal tissues ( Fig. 2e ). Together, these data indicate that RSPO2 expression is downregulated in the majority of CRC tumours due to promoter hypermethylation. 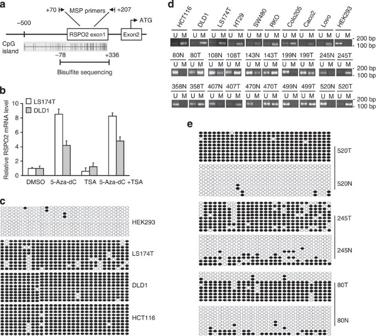Figure 2: The RSPO2 promoter is hypermethylated in CRC cells and tumours. (a) Schematic representation of the CpG island in the RSPO2 promoter region. Vertical bars indicate the location of the CpG sites. Arrows indicate the position of primers for MSP. Positions −78 to +336 indicate the region that was sequenced by bisulphite sequencing PCR. (b) RSPO2 expression reactivation. Cells were treated with 5 μM 5-aza-2'-deoxycytidine (5-Aza-dC) for 3 days and/or 0.3 μM trichostatin A (TSA) for 1 day, and the RSPO2 mRNA level was determined using qRT−PCR. Error bars indicate s.d. of three independent experiments. (c) Bisulphite sequencing of the RSPO2 promoter in HEK293 and CRC cell lines. Open and filled circles represent unmethylated and methylated CpG sites, respectively. Each row represents a single clone. (d) Methylation analysis of RSPO2 in CRC cells, primary tumours (T) and matched normal mucosa (N) by MSP using primers specific for methylated (M) or unmethylated (U) templates. (e) Bisulphite sequencing of primary CRC tumours (T) and matched normal mucosa (N). Error bars indicate the s.d. Figure 2: The RSPO2 promoter is hypermethylated in CRC cells and tumours. ( a ) Schematic representation of the CpG island in the RSPO2 promoter region. Vertical bars indicate the location of the CpG sites. Arrows indicate the position of primers for MSP. Positions −78 to +336 indicate the region that was sequenced by bisulphite sequencing PCR. ( b ) RSPO2 expression reactivation. Cells were treated with 5 μM 5-aza-2'-deoxycytidine (5-Aza-dC) for 3 days and/or 0.3 μM trichostatin A (TSA) for 1 day, and the RSPO2 mRNA level was determined using qRT−PCR. Error bars indicate s.d. of three independent experiments. ( c ) Bisulphite sequencing of the RSPO2 promoter in HEK293 and CRC cell lines. Open and filled circles represent unmethylated and methylated CpG sites, respectively. Each row represents a single clone. ( d ) Methylation analysis of RSPO2 in CRC cells, primary tumours (T) and matched normal mucosa (N) by MSP using primers specific for methylated (M) or unmethylated (U) templates. ( e ) Bisulphite sequencing of primary CRC tumours (T) and matched normal mucosa (N). Error bars indicate the s.d. Full size image RSPO2 has an inhibitory effect on CRC cell growth The prevalence of RSPO2 downregulation raises an intriguing possibility that RSPO2 silencing may be not only a cancer-specific signature but also a cancer-promoting event in CRCs. Indeed, we found that increasing the expression of RSPO2 in two different CRC cell lines, LS174T and DLD1, suppressed cell proliferation ( Fig. 3a,b ). Among the four recombinant human R-spondin proteins we examined, only RSPO2 dose-dependently inhibited the growth of both CRC cell lines ( Fig. 3c and Supplementary Fig. 2 ). Conversely, depletion of RSPO2 by short interfering RNA (siRNA) treatment in RSPO2-overexpressing LS174T and DLD1 cells resulted in a significant enhancement of cell proliferation in both cell lines ( Fig. 3d and Supplementary Fig. 3 ). Likewise, the tumour development for derivatives of LS174T, DLD1 and HCT116 that ectopically overexpressed RSPO2 was also much slower than for the respective parental cell lines ( Fig. 3e,f and Supplementary Fig. 4 ). Taken together, our data demonstrate that RSPO2 can inhibit CRC cell growth both in vitro and in vivo . These results strongly suggest that RSPO2 functions as a tumour suppressor in these CRC cells. 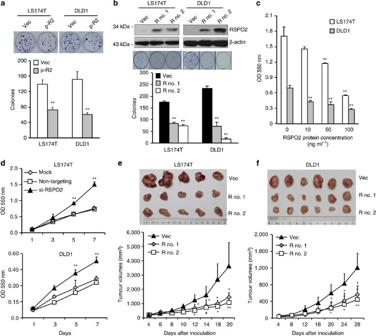Figure 3:RSPO2 suppresses CRC tumour growth. (a) RSPO2 colony formation-suppressing activity. The numbers of G418-resistant colonies that arose from transfection with the RSPO2 expression vector (p-R2) or the control empty expression vector pcDNA3.1 (Vec) are shown. Error bars indicate s.d. of three independent experiments. **P<0.01 versus Vec. (b) Clonogenic assay in CRC cells that stably overexpress RSPO2. Two randomly picked stable RSPO2-overexpressing clones (R no. 1 and R no. 2) and a control clone with empty vector (Vec) were used for the experiments. The RSPO2 protein level was determined using western blotting (top). Error bars indicate s.d. of three independent experiments. **P<0.01 versus Vec. (c) MTT assay with CRC cells treated with recombinant RSPO2 protein for 3 days. Data were calculated from triplicates. **P<0.01 versus group zero. (d) MTT assay in CRC cells following siRNA-mediated RSPO2 (si-RSPO2) knockdown. Stable RSPO2-overexpressing clones R no. 1 of both LS174T and DLD1 inFig. 3bwere used for the experiment. Data were calculated from triplicates. **P<0.01 versus non-targeting. (e,f) RSPO2 suppresses CRC tumorigenicityin vivo. Subcutaneous tumour regeneration with LS174T and DLD1 cells was assessed in nude mice. The volume of the generated tumours was measured during the indicated period (bottom), and photographs of the tumours at autopsy are presented (top). Error bars indicate s.d. of the tumour volume (n=5–6). *P<0.05 versus Vec; **P<0.01 versus Vec. (a–f) Mean±s.d.; statistical significance was determined by Student’st-test. Figure 3: RSPO2 suppresses CRC tumour growth . ( a ) RSPO2 colony formation-suppressing activity. The numbers of G418-resistant colonies that arose from transfection with the RSPO2 expression vector (p-R2) or the control empty expression vector pcDNA3.1 (Vec) are shown. Error bars indicate s.d. of three independent experiments. ** P <0.01 versus Vec. ( b ) Clonogenic assay in CRC cells that stably overexpress RSPO2. Two randomly picked stable RSPO2-overexpressing clones (R no. 1 and R no. 2) and a control clone with empty vector (Vec) were used for the experiments. The RSPO2 protein level was determined using western blotting (top). Error bars indicate s.d. of three independent experiments. ** P <0.01 versus Vec. ( c ) MTT assay with CRC cells treated with recombinant RSPO2 protein for 3 days. Data were calculated from triplicates. ** P <0.01 versus group zero. ( d ) MTT assay in CRC cells following siRNA-mediated RSPO2 (si-RSPO2) knockdown. Stable RSPO2-overexpressing clones R no. 1 of both LS174T and DLD1 in Fig. 3b were used for the experiment. Data were calculated from triplicates. ** P <0.01 versus non-targeting. ( e , f ) RSPO2 suppresses CRC tumorigenicity in vivo . Subcutaneous tumour regeneration with LS174T and DLD1 cells was assessed in nude mice. The volume of the generated tumours was measured during the indicated period (bottom), and photographs of the tumours at autopsy are presented (top). Error bars indicate s.d. of the tumour volume ( n =5–6). * P <0.05 versus Vec; ** P <0.01 versus Vec. ( a – f ) Mean±s.d. ; statistical significance was determined by Student’s t -test. Full size image RSPO2 has an inhibitory effect on Wnt signaling in CRC cells The suggestion that RSPO2 functions as a growth suppressor is perplexing because R-spondins are Wnt agonists and thus should promote growth. This contradictory observation prompted us to consider that the growth-suppressive effect of RSPO2 may be a unique feature in CRC cells. Indeed, we found that while RSPO2 enhanced β-catenin reporter activity in HEK293 cells ( Supplementary Fig. 5a,b ), as shown previously [30] , it had an antagonistic effect on β-catenin reporter activity in CRC cell lines. In LS174T, DLD1 and HCT116 cells, exogenous RSPO2 overexpression or recombinant protein stimulation decreased β-catenin reporter activity in a dose-dependent manner ( Fig. 4a and Supplementary Fig. 6 ). In contrast, RSPO2 had no effect on the activity of FopFlash, a negative control β-catenin reporter ( Supplementary Fig. 7 ). In addition, depleting RSPO2 by siRNA knockdown increased β-catenin reporter activity ( Fig. 4b ). These data indicate that, although RSPO2 can function as a Wnt agonist in HEK293 cells, it has an inhibitory effect of Wnt signaling in CRC cell lines. 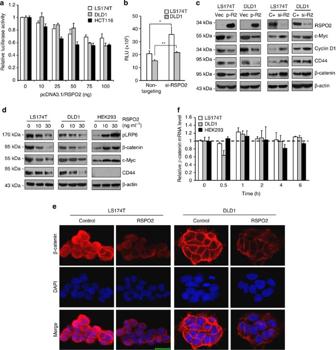Figure 4: RSPO2 suppresses Wnt/β-catenin signaling in CRC cells. (a) β-catenin reporter assay in three CRC cell lines following RSPO2 overexpression. Error bars indicate s.d. of three independent experiments. (b) β-catenin reporter assay in response to RSPO2 knockdown. Stable RSPO2-overexpressing clones of both LS174T and DLD1 cells were used for si-RSPO2 knockdown. A non-targeting siRNA was used as a control. Error bars indicate s.d. of three independent experiments. Statistical significance was determined by Student’st-test. *P<0.05; **P<0.01. (c) The effect of RSPO2 on Wnt target gene expression. For RSPO2 overexpression (left panel), cells were transiently transfected with either the RSPO2 overexpression vector (p-R2) or the control vector pcDNA3.1 (Vec). For RSPO2 knockdown (right panel), stable clones R no. 1 of both LS174T and DLD1 inFig. 3bwere used for si-RSPO2 (si-R2) knockdown. A non-targeting siRNA was used as a control (C+). (d) The effect of RSPO2 protein exposure on phosphorylated LRP6 (pLRP6), c-Myc, CD44 and β-catenin accumulation. Cells were treated with 0, 10 or 30 ng ml−1RSPO2 protein for 5 h. (e) RSPO2-induced β-catenin changes in CRC cells. Cells were stimulated without (Control) or with RSPO2 (40 ng ml−1) for 5 h. β-Catenin was detected using immunofluorescence staining and confocal microscopy. Scale bar: 20 μm. (f)β-cateninmRNA levels in response to RSPO2 treatment. Cells were stimulated with 40 ng ml−1RSPO2, and β-catenin mRNA levels were determined using qRT–PCR. Error bars indicate s.d. of three independent experiments. Figure 4: RSPO2 suppresses Wnt/β-catenin signaling in CRC cells. ( a ) β-catenin reporter assay in three CRC cell lines following RSPO2 overexpression. Error bars indicate s.d. of three independent experiments. ( b ) β-catenin reporter assay in response to RSPO2 knockdown. Stable RSPO2-overexpressing clones of both LS174T and DLD1 cells were used for si-RSPO2 knockdown. A non-targeting siRNA was used as a control. Error bars indicate s.d. of three independent experiments. Statistical significance was determined by Student’s t -test. * P <0.05; ** P <0.01. ( c ) The effect of RSPO2 on Wnt target gene expression. For RSPO2 overexpression (left panel), cells were transiently transfected with either the RSPO2 overexpression vector (p-R2) or the control vector pcDNA3.1 (Vec). For RSPO2 knockdown (right panel), stable clones R no. 1 of both LS174T and DLD1 in Fig. 3b were used for si-RSPO2 (si-R2) knockdown. A non-targeting siRNA was used as a control (C+). ( d ) The effect of RSPO2 protein exposure on phosphorylated LRP6 (pLRP6), c-Myc, CD44 and β-catenin accumulation. Cells were treated with 0, 10 or 30 ng ml −1 RSPO2 protein for 5 h. ( e ) RSPO2-induced β-catenin changes in CRC cells. Cells were stimulated without (Control) or with RSPO2 (40 ng ml −1 ) for 5 h. β-Catenin was detected using immunofluorescence staining and confocal microscopy. Scale bar: 20 μm. ( f ) β-catenin mRNA levels in response to RSPO2 treatment. Cells were stimulated with 40 ng ml −1 RSPO2, and β-catenin mRNA levels were determined using qRT–PCR. Error bars indicate s.d. of three independent experiments. Full size image The antagonistic effect of RSPO2 on Wnt signaling offers a plausible explanation for its growth-suppressive effect in CRC cells. To verify this possibility, we examined the expression of several key Wnt target genes, such as c-Myc , Cyclin D1 and CD44 , which are tightly associated with CRC cell proliferation and tumorigenesis [32] . We found that the ectopic overexpression of RSPO2 in both LS174T and DLD1 cells resulted in significant reductions in the levels of these Wnt target genes ( Fig. 4c ). Conversely, the knockdown of RSPO2 in these cell lines led to significant increases in the expression levels of these genes ( Fig. 4c ). More importantly, we found that the levels of phosphorylated LRP6 and cytosolic β-catenin were reduced in LS174T and DLD1 cells but increased in HEK293 cells following RSPO2 protein treatments ( Fig. 4d,e ). The changes in β-catenin accumulation were not associated with significant alterations in its mRNA levels ( Fig. 4f ); therefore, it appears that RSPO2 suppresses Wnt signaling by reducing the accumulation of β-catenin in CRC cells. RSPO2 causes a unique LGR5-dependent attenuation of Wnt signaling Previously, RSPO2 was described as an oncogene in human CRCs due to its role in β-catenin reporter activation in the HT29 cell line [29] . Here we confirmed that RSPO2 specifically promotes Wnt signaling in HT29 cell ( Fig. 5a–d ). We found that HT29 was the only tested CRC cell line in which Wnt signaling was enhanced by R-spondins, including RSPO1, 2 and 3 ( Fig. 5e and Supplementary Figs 6 and 8 ). RSPO2 overexpression promoted HT29 cell growth and RSPO2 knockdown showed the opposite effect ( Fig. 5f,g ); these results indicated that RSPO2 indeed functions as an oncogene in HT29 cells. The contradictory phenotypes in HT29 and other CRC cell lines suggest that distinct features characteristic to each cell line dictate the discrepant response to RSPO2. To explore this possibility, we performed a time course study in HT29 cells and found that RSPO2 caused a progressive increase in both LRP6 phosphorylation and β-catenin accumulation ( Fig. 6a ). However, the same treatment in LS174T or DLD1 cells resulted in distinct biphasic effects ( Fig. 6a ). Specifically, RSPO2 caused an initial induction of LRP6 phosphorylation and β-catenin accumulation within the first hour after the treatment, which was followed by an attenuated response thereafter. The levels of cytosolic β-catenin and c-Myc at the later time points were lower than the levels prior to the treatment ( Fig. 6a ). The biphasic response suggests that a Wnt feedback mechanism exists in these CRC cells. As this work was in progress, de Lau et al . [11] reported that RSPO2 is the ligand for LGRs, including LGR5 (refs 10 , 11 ). Coincidentally, LGR5 is a known Wnt target gene in CRC cell lines [32] . These findings led us to consider that LGR5 may be involved in the RSPO2-induced Wnt signaling attenuation. Indeed, we found that the LGR5 mRNA and protein levels were transiently elevated in both LS174T and DLD1 cells upon RSPO2 stimulation ( Fig. 6b,c ). However, the same RSPO2 treatment did not lead to an apparent LGR5 elevation in HT29 or HEK293 cells ( Fig. 6b and Supplementary Fig. 9 ). Furthermore, RSPO2 stimulation clearly increased the expression of LGR5 in HCT116 cells, which, like HT29 and HEK293 cells, express almost undetectable levels of endogenous LGR5 ( Supplementary Fig. 10 ) [11] . The elevated LGR5 expression exclusively occurs in the CRC cells that showed attenuated Wnt signaling and tumour growth potential; these results suggest that the distinctive effects of RSPO2 may be related to the status of LGR5 expression following RSPO2 treatment. 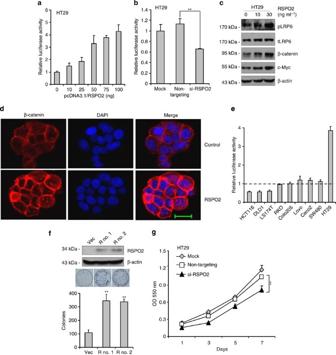Figure 5: RSPO2 promotes Wnt signaling and tumour cell growth in CRC HT29 cells. (a) β-catenin reporter assay in HT29 cells with RSPO2 overexpression. Error bars indicate s.d. of three independent experiments. (b) β-catenin reporter assay in HT29 cells following RSPO2 knockdown. HT29 cells were transfected with either targeting siRNA (si-RSPO2) or non-targeting siRNA. Cells subjected to the transfection procedure in the absence of siRNA were set as mock-treated control (Mock). Error bars indicate s.d. of three independent experiments. **P<0.01 versus non-targeting group. (c) The effect of RSPO2 protein exposure on the accumulation of endogenous Wnt signaling proteins. HT29 cells were treated with 0, 10 or 30 ng ml−1RSPO2 protein for 5 h. (d) RSPO2-induced cytosolic and nuclear β-catenin changes in HT29 cells. Cells were stimulated without (Control) or with RSPO2 (40 ng ml−1) for 5 h. β-Catenin was detected using immunofluorescence staining and confocal microscopy. Scale bar: 20 μm. (e) β-catenin reporter assay in nine CRC cell lines following RSPO2 overexpression. Data were calculated from triplicates. (f) RSPO2 promotes HT29 CRC tumour cell growth. The clonogenic assay was performed on two randomly selected stable RSPO2-overexpressing clones (R no. 1 and R no. 2) and an empty vector control (Vec). The RSPO2 protein level was determined using western blotting (top). Error bars indicate s.d. of three independent experiments. **P<0.01 versus Vec. (g) The effects of RSPO2 knockdown on HT29 cell proliferation. Data were calculated from triplicates. **P<0.01 versus non-targeting group. (b,f,g) Mean±s.d.; statistical significance was determined by Student’st-test. Figure 5: RSPO2 promotes Wnt signaling and tumour cell growth in CRC HT29 cells. ( a ) β-catenin reporter assay in HT29 cells with RSPO2 overexpression. Error bars indicate s.d. of three independent experiments. ( b ) β-catenin reporter assay in HT29 cells following RSPO2 knockdown. HT29 cells were transfected with either targeting siRNA (si-RSPO2) or non-targeting siRNA. Cells subjected to the transfection procedure in the absence of siRNA were set as mock-treated control (Mock). Error bars indicate s.d. of three independent experiments. ** P <0.01 versus non-targeting group. ( c ) The effect of RSPO2 protein exposure on the accumulation of endogenous Wnt signaling proteins. HT29 cells were treated with 0, 10 or 30 ng ml −1 RSPO2 protein for 5 h. ( d ) RSPO2-induced cytosolic and nuclear β-catenin changes in HT29 cells. Cells were stimulated without (Control) or with RSPO2 (40 ng ml −1 ) for 5 h. β-Catenin was detected using immunofluorescence staining and confocal microscopy. Scale bar: 20 μm. ( e ) β-catenin reporter assay in nine CRC cell lines following RSPO2 overexpression. Data were calculated from triplicates. ( f ) RSPO2 promotes HT29 CRC tumour cell growth. The clonogenic assay was performed on two randomly selected stable RSPO2-overexpressing clones (R no. 1 and R no. 2) and an empty vector control (Vec). The RSPO2 protein level was determined using western blotting (top). Error bars indicate s.d. of three independent experiments. ** P <0.01 versus Vec. ( g ) The effects of RSPO2 knockdown on HT29 cell proliferation. Data were calculated from triplicates. ** P <0.01 versus non-targeting group. ( b , f , g ) Mean±s.d. ; statistical significance was determined by Student’s t -test. 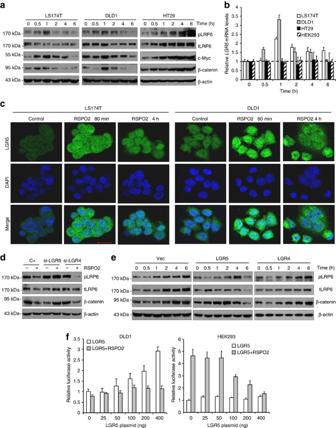Figure 6: RSPO2-induced Wnt signaling suppression is LGR5-dependent. (a) Time course of Wnt pathway protein levels following RSPO2 treatment. Cells were stimulated with RSPO2 (40 ng ml−1) for 0–6 h, and phosphorylated LRP6 (pLRP6), total LRP6 (tLRP6), c-Myc and cytosolic β-catenin were probed using western blotting. (b) LGR5 mRNA levels in response to RSPO2 treatment. Cells were stimulated with RSPO2 (40 ng ml−1) for 0−6 h. LGR5 mRNA levels were determined using qRT–PCR. Error bars indicate the s.d. of three independent experiments. (c) The effect of RSPO2 exposure on LGR5 protein expression. Cells were stimulated without (Control) or with RSPO2 (40 ng ml−1) for 80 min or 4 h. LGR5 protein was detected using immunofluorescence staining and confocal microscopy. Scale bar: 20 μm. (d) LGR5 knockdown attenuated RSPO2-induced Wnt signaling suppression in CRC cells. DLD1 cells were transfected with either non-targeting siRNA (C+) or siRNA targeting LGR4 (si-LGR4) or LGR5 (si-LGR5), and 2 days later, the cells were stimulated with RSPO2 (40 n ml−1) for 5 h. (e) Overexpression of LGR5 reversed RSPO2-induced Wnt signaling activation in HEK293 cells. HEK293 cells stably overexpressing LGR4, LGR5 or empty vector (Vec) were stimulated with RSPO2 (40 ng ml−1) for 0–6 h in DMEM with 1% FBS. (f) The effects of LGR5 and RSPO2 co-transfection on β-catenin reporter activity. A quantity of 100 ng of RSPO2 expression plasmid was used. Error bars indicate the s.d. of three independent experiments. Full size image Figure 6: RSPO2-induced Wnt signaling suppression is LGR5-dependent. ( a ) Time course of Wnt pathway protein levels following RSPO2 treatment. Cells were stimulated with RSPO2 (40 ng ml −1 ) for 0–6 h, and phosphorylated LRP6 (pLRP6), total LRP6 (tLRP6), c-Myc and cytosolic β-catenin were probed using western blotting. ( b ) LGR5 mRNA levels in response to RSPO2 treatment. Cells were stimulated with RSPO2 (40 ng ml −1 ) for 0−6 h. LGR5 mRNA levels were determined using qRT–PCR. Error bars indicate the s.d. of three independent experiments. ( c ) The effect of RSPO2 exposure on LGR5 protein expression. Cells were stimulated without (Control) or with RSPO2 (40 ng ml −1 ) for 80 min or 4 h. LGR5 protein was detected using immunofluorescence staining and confocal microscopy. Scale bar: 20 μm. ( d ) LGR5 knockdown attenuated RSPO2-induced Wnt signaling suppression in CRC cells. DLD1 cells were transfected with either non-targeting siRNA (C+) or siRNA targeting LGR4 (si-LGR4) or LGR5 (si-LGR5), and 2 days later, the cells were stimulated with RSPO2 (40 n ml −1 ) for 5 h. ( e ) Overexpression of LGR5 reversed RSPO2-induced Wnt signaling activation in HEK293 cells. HEK293 cells stably overexpressing LGR4, LGR5 or empty vector (Vec) were stimulated with RSPO2 (40 ng ml −1 ) for 0–6 h in DMEM with 1% FBS. ( f ) The effects of LGR5 and RSPO2 co-transfection on β-catenin reporter activity. A quantity of 100 ng of RSPO2 expression plasmid was used. Error bars indicate the s.d. of three independent experiments. Full size image To verify the role of LGR5 in RSPO2-induced Wnt signaling attenuation, we knocked down LGR5 in DLD1 cells. We found that the siRNA-mediated depletion of LGR5 (but not LGR4) restored the attenuated LRP6 phosphorylation and β-catenin accumulation induced by RSPO2 ( Fig. 6d and Supplementary Fig. 11 ). These data indicate that LGR5 plays an essential role in RSPO2-induced Wnt signaling attenuation. To confirm the specificity of LGR5 in Wnt signaling regulation, we constructed cell lines that stably overexpress LGR5 or LGR4 ( Supplementary Fig. 12 ). We found that the ectopic stable overexpression of LGR5 in HEK293 cells was sufficient to attenuate the stimulatory effect of RSPO2 on Wnt signaling. The significantly increased LRP6 phosphorylation and β-catenin accumulation were reversed in LGR5-overexpressing HEK293 cells at a later 6-h time point ( Fig. 6e ). Although RSPO2 or LGR5 alone activated the β-catenin reporter in HEK293 or DLD1 cells, respectively, the co-transfection of LGR5 and RSPO2 clearly attenuated the elevated reporter activity in both cell lines ( Fig. 6f ). Together, these data indicate that the suppression of Wnt signaling by RSPO2 is LGR5-dependent. Specifically, in CRC cells that express high levels of LGR5 following RSPO2 treatment, RSPO2 negatively regulates Wnt/β-catenin signaling and suppresses tumour cell growth. RSPO2 suppresses Wnt signaling by stabilizing ZNRF3 To confirm that LGR5-dependent Wnt/β-catenin signaling attenuation suppresses CRC cell growth induced by RSPO2, we constructed a stable LGR5-expressing HT29 cell line ( Fig. 5 and Supplementary Fig. 12 ). We found that the overexpression of LGR5 directly reversed the activation of Wnt signaling induced by RSPO2 ( Fig. 7a ). Furthermore, the RSPO2-induced cell growth promotion was retarded, and the combination of RSPO2 and LGR5 conversely suppressed the HT29 cell growth. These data indicate that LGR5 specifically functions in RSPO2-induced tumour suppression. Interestingly, we also observed that the overexpression of LGR5 alone inhibited HT29 cell proliferation ( Fig. 7b,c ), which supports the hypothesis that LGR5 is a negative regulator of CRC tumourigenicity as reported previously [33] , [34] . To explore the association between Wnt signaling regulation and the RSPO2–LGR5 interaction, we investigated the levels of the cell-surface transmembrane E3 ubiquitin ligase ZNRF3 following RSPO2 treatment. In DLD1 and LS174T cells, RSPO2 markedly increased the level of membrane-associated ZNRF3, but not the level in the total cell lysate ( Fig. 7d ). ZNRF3 is a negative Wnt signaling modulator that functions by promoting the degradation of the Wnt receptor LRP6 (ref. 35 ). Consistent with this activity, RSPO2 decreased the LRP6 levels in both DLD1 and LS174T cell lines ( Fig. 6a ). Together, these results suggest that RSPO2 suppresses Wnt signaling by stabilizing the membrane-associated ZNRF3. In HT29 cells that do not express LGR5, RSPO2 decreased the level of membrane-associated ZNRF3 ( Fig. 7e ). Conversely, the combination of LGR5 and RSPO2 increased the accumulation of ZNRF3 at the cell membrane ( Fig. 7e ). These data suggest that RSPO2 interacts with LGR5 to stabilize ZNRF3 on the cell membrane. 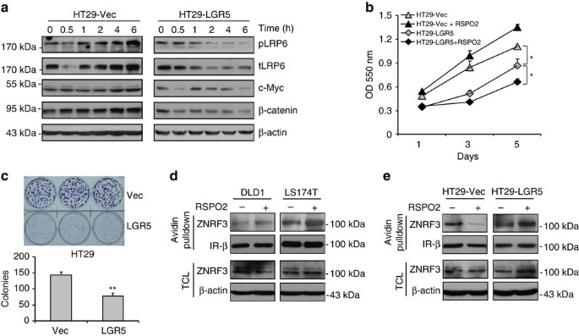Figure 7: RSPO2 interacts with LGR5 to stabilize ZNRF3 in CRC cells. (a) The effect of LGR5 on RSPO2-induced Wnt signaling activation. HT29 cells stably overexpressing LGR5 (HT29-LGR5) or empty vector (HT29-Vec) were stimulated with RSPO2 (40 ng ml−1) for 0–6 h. (b) The effect of LGR5 on RSPO2-induced cell proliferation. HT29 cells stably expressing LGR5 (HT29-LGR5) or empty vector (HT29-Vec) were treated without or with 40 ng ml−1RSPO2, and the cell numbers were determined by the MTT assay. The LGR5 protein level was determined using western blotting (Supplementary Fig. 12). Data were calculated from triplicates. *P<0.05. (c) Clonogenic assay in HT29 cells that stably overexpress LGR5. A stable LGR5-overexpressing clone (LGR5) and a control clone with empty vector (Vec) were used for experiments. Error bars indicate s.d. of three independent experiments. **P<0.01. (d) RSPO2 increases the level of membrane-associated ZNRF3 in CRC cells. Cells were stimulated with 40 ng ml−1RSPO2 for 6 h, and the total cell lysate (TCL) and the membrane protein (avidin pull-down) were probed using western blotting. (e) LGR5 promotes RSPO2-induced membrane-associated ZNRF3 turnover. HT29 cells stably overexpressing LGR5 (HT29-LGR5) or empty vector (HT29-Vec) were stimulated with 40 ng ml−1RSPO2 for 6 h. (b,c) Mean±s.d.; statistical significance was determined using Student’st-test. Figure 7: RSPO2 interacts with LGR5 to stabilize ZNRF3 in CRC cells. ( a ) The effect of LGR5 on RSPO2-induced Wnt signaling activation. HT29 cells stably overexpressing LGR5 (HT29-LGR5) or empty vector (HT29-Vec) were stimulated with RSPO2 (40 ng ml −1 ) for 0–6 h. ( b ) The effect of LGR5 on RSPO2-induced cell proliferation. HT29 cells stably expressing LGR5 (HT29-LGR5) or empty vector (HT29-Vec) were treated without or with 40 ng ml −1 RSPO2, and the cell numbers were determined by the MTT assay. The LGR5 protein level was determined using western blotting ( Supplementary Fig. 12 ). Data were calculated from triplicates. * P <0.05. ( c ) Clonogenic assay in HT29 cells that stably overexpress LGR5. A stable LGR5-overexpressing clone (LGR5) and a control clone with empty vector (Vec) were used for experiments. Error bars indicate s.d. of three independent experiments. ** P <0.01. ( d ) RSPO2 increases the level of membrane-associated ZNRF3 in CRC cells. Cells were stimulated with 40 ng ml −1 RSPO2 for 6 h, and the total cell lysate (TCL) and the membrane protein (avidin pull-down) were probed using western blotting. ( e ) LGR5 promotes RSPO2-induced membrane-associated ZNRF3 turnover. HT29 cells stably overexpressing LGR5 (HT29-LGR5) or empty vector (HT29-Vec) were stimulated with 40 ng ml −1 RSPO2 for 6 h. ( b , c ) Mean±s.d. ; statistical significance was determined using Student’s t -test. Full size image Correlation between RSPO2 and LGR5 expression in CRC tumours The constitutive activation of Wnt signaling is present in the majority of human CRCs, and the upregulation of LGR5 is also commonly observed in clinical CRC samples ( Supplementary Fig. 13 ) [36] . Based on our feedback hypothesis, we predicted that the expression levels of RSPO2 and LGR5 would correlate in primary CRC tumours. Indeed, we observed a significant inverse correlation between downregulated RSPO2 and elevated LGR5 expression (Spearman P <0.001, n =80) ( Fig. 8a ). Notably, among the 80 pairs of CRC samples, only one tumour sample (Case no. 125) showed significantly increased RSPO2 expression (more than twofold). Upon further investigation of this sample, we found that the upregulation of RSPO2 was due to a recurrent gene fusion of RSPO2 and EIF3E ( Supplementary Fig. 14 ), which was reported previously [29] . Moreover, sequencing analysis showed that a G to A mutation occurred within the only TCF-binding site in the promoter of the LGR5 gene ( Fig. 8b ); this mutation is consistent with the significantly downregulated (~32-fold) LGR5 expression. In addition, while Wnt3a stimulation increased both c-Myc and LGR5 expression in LS174T cells, it increased c-Myc but not LGR5 expression in HT29 cells ( Fig. 8c ). These data indicate that in a few CRC cell lines or tumours, promoter mutations or cellular context difference may impair LGR5 expression, and thus disrupt the formation of the RSPO2–LGR5-mediated Wnt signaling feedback loop. 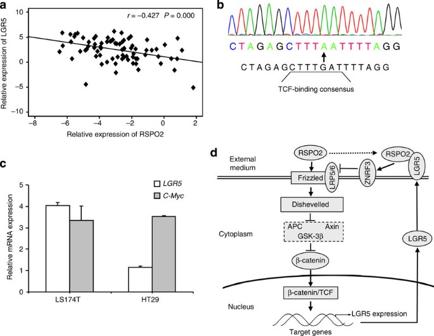Figure 8: Correlation betweenRSPO2and LGR5 expression in CRC primary tumours. (a) Correlation analysis of RSPO2 and LGR5 expression in human CRC tumour samples. There was a negative correlation between RSPO2 and LGR5 expression (n=80, Spearman’sP<0.001). (b) A mutation from G to A occurred within the TCF-binding site of the LGR5 promoter in Case no. 125 CRC tumour sample, as determined by Sanger sequencing. (c) Wnt target geneLGR5and c-Myc expressions in response to Wnt3a stimulation. Cells were stimulated with Wnt3a (100 ng ml−1) for 12 h, LGR5 and c-Myc mRNA levels were determined using qRT–PCR. Error bars indicate s.d. of three independent experiments. (d) Scheme of the negative feedback loop of Wnt/β-catenin pathway induced by RSPO2 and LGR5. Figure 8: Correlation between RSPO2 and LGR5 expression in CRC primary tumours. ( a ) Correlation analysis of RSPO2 and LGR5 expression in human CRC tumour samples. There was a negative correlation between RSPO2 and LGR5 expression ( n =80, Spearman’s P <0.001). ( b ) A mutation from G to A occurred within the TCF-binding site of the LGR5 promoter in Case no. 125 CRC tumour sample, as determined by Sanger sequencing. ( c ) Wnt target gene LGR5 and c-Myc expressions in response to Wnt3a stimulation. Cells were stimulated with Wnt3a (100 ng ml −1 ) for 12 h, LGR5 and c-Myc mRNA levels were determined using qRT–PCR. Error bars indicate s.d. of three independent experiments. ( d ) Scheme of the negative feedback loop of Wnt/β-catenin pathway induced by RSPO2 and LGR5. Full size image R-spondins were first discovered as secreted Wnt agonists [30] . Given the crucial role of Wnt signaling in tumorigenesis, R-spondins have been considered potential oncogenes. In support of this presumption, rare disruptions of the RSPO1 gene in humans cause a predisposition to skin carcinoma [13] , and RSPO3 promotes the tumorigenicity of mammary epithelial cells in mice [19] . A deficiency for RSPO2 in mice is postnatally lethal, suggesting that RSPO2 has functions that are non-redundant from the other R-spondin members [24] . In this study, we demonstrated that RSPO2 inhibited CRC tumour growth both in vitro and in vivo . Our data strongly suggest that RSPO2 functions as a tumour suppressor in most human CRC tumours. This finding indicates that R-spondins can function either as oncogenes or as tumour suppressors depending on the type of cancer. In three CRC cell lines, we demonstrated that RSPO2 treatment attenuated Wnt signaling and eventually suppressed the growth of CRC tumour cells. The DLD1 cell line has an Apc truncation; LS174T and HCT116 cells have β-catenin mutations. We showed that restoring of RSPO2 attenuated Wnt signaling even in the presence of downstream mutations. This result is similar to the function of a known Wnt antagonist family, the secreted frizzled related proteins [37] . Furthermore, we found that the repression of Wnt signaling by RSPO2 was LGR5-dependent and occurred exclusively in CRC cells that expressed high levels of LGR5 following RSPO2 treatment. Based on our results and previous reports describing LGR5 as the ligand for RSPO2 and as a known Wnt target gene in CRC cells [11] , [32] , we propose a novel RSPO2-induced Wnt signaling feedback model ( Fig. 8d ). In this model, RSPO2 enables a transient activation of the Wnt pathway and a pronounced upregulation of LGR5 expression, which in turn interacts with RSPO2 to stabilize membrane-associated ZNRF3, and thus promotes LRP6 degradation. These alterations create a negative feedback loop that attenuates β-catenin accumulation and Wnt target gene expression and eventually exerts a net growth-suppressive effect on CRC cells. In the majority of human CRCs, Wnt signaling is constitutively activated, and the expression of LGR5 is upregulated [36] . In such a cellular context, according to the feedback mechanism we propose, RSPO2 downregulation would favour tumour cell growth; this is precisely the outcome of RSPO2 expression that we observed in clinical CRC samples ( Fig. 1 ). Further supporting this hypothesis, we observed an inverse correlation between RSPO2 and LGR5 expression in clinical CRC samples ( Fig. 8a ). The fact that RSPO2 is expressed in normal crypt epithelia but is silenced in the vast majority of CRCs argues that RSPO2 acts primarily as a tumour suppressor in human colonic epithelia. The exception to this is that in a few CRC cell lines, such as HT29, or in tumours that are deficient for LGR5 expression due to promoter mutation or cellular context differences, RSPO2 constitutively promoted Wnt signaling and functioned as an oncogene. Here we have identified a unique role of LGR5 in the suppression of Wnt signaling by RSPO2 in CRC cells. We also investigated the preliminary mechanism of how the interaction of RSPO2 and LGR5 leads to the modulation of Wnt/β-catenin signaling. In CRC cells, we demonstrated that RSPO2 promoted total LRP6 degradation and simultaneously repressed LRP6 phosphorylation and β-catenin accumulation. LRP6 phosphorylation is crucial for β-catenin stabilization, and both are hallmark indicators of Wnt pathway activation [38] . We found that co-stimulation with RSPO2 and LGR5 promoted LRP6 degradation, and that the attenuation of Wnt signaling by RSPO2 was LGR5-dependent. Our results are consistent with the finding in HEK293 cells that the co-expression of LGR5 with LRP6 increases LRP6 internalization and enhances LRP6 degradation following RSPO2 stimulation [39] . We also demonstrated that RSPO2 increased the accumulation of membrane-associated ZNRF3 in CRC cells and that LGR5 was essential for this process. ZNRF3 is a tumour suppressor and a negative Wnt signaling modulator that promotes the degradation of LRP6 (refs 35 , 40 ). More recently, the physical linkage of R-spondin with LGRs was confirmed by their structural analysis [41] , [42] , [43] . Our data, together with these previous findings, suggest that RSPO2 interacts with LGR5 to stabilize the membrane-associated ZNRF3, thus decreasing LRP6 accumulation and phosphorylation, and eventually interfering with both the β-catenin accumulation and Wnt signaling activation. The interaction between RSPO1 and LGR4 induces the clearance of ZNRF3 from the membrane [35] . In our study, the interaction of RSPO2 and LGR5 resulted in membrane-associated ZNRF3 accumulation. These contradictory results suggest that LGR4 and LGR5 may have antagonistic effects on Wnt signaling regulation as reported [44] . Further studies are needed to address this possibility. Previous reports showed that LGR5 and R-spondins mediate a synergistic activation of Wnt signaling [10] , [11] , [12] . It is noteworthy that those results were only observed in HEK293T cells with β-catenin reporter assays. In CRC cells, we demonstrated that the RSPO2-induced Wnt signaling turnover is LGR5-dependent. In our study, the RSPO2–LGR5-mediated Wnt signaling attenuation was evidenced by the reduction of β-catenin accumulation and Wnt target gene expression. The co-expression of LGR5 with RSPO2 eventually suppressed Wnt signaling activation, supporting the finding that LGR5 is a negative regulator of the Wnt pathway in the intestine [33] , [34] . Similar to our data, Carmon et al . [10] found that RSPO1 leads to β-catenin reduction in LGR5-overexpressing HEK293T cells, and this phenomenon is in contrast with their β-catenin reporter assay. One possible explanation they provided was that RSPO1 stimulation induced a transient increase in β-catenin that led to a rapid increase in reporter gene transcription and an accumulation of abundant reporter enzyme activity. A more recent report also showed that the stimulation of LGR5-overexpressing corneal endothelial cells with RSPO1 accelerated phosphorylated LRP6 degradation and β-catenin turnover [45] . Furthermore, in our study, the co-transfection of LGR5 and RSPO2 attenuated the elevated reporter activity in both HEK293 and DLD1 cell lines ( Fig. 6f ). It should be noted that our β-catenin reporter assay was performed 48 h after co-transfection. When we conducted the assay at 36 h, we did not see the inhibitory effects. These results suggest that the genuine Wnt signaling turnover could be obscured if it was only observed with β-catenin reporter assay. The aberrant methylation of CpG-rich sequences is a common epigenetic change in human cancers. The methylation of R-spondin members has been reported. CpG islands in the promoter of the RSPO1 gene are hypermethylated in human leukaemia cells and cancer patients [46] . RSPO4 shows aberrant DNA methylation in human oesophageal squamous carcinoma [47] . In this study, we found that aberrant methylation of the RSPO2 gene occurred in >75% of primary colorectal carcinomas and that the restoration of RSPO2 expression inhibited CRC cell growth; these results suggest that the aberrant methylation of RSPO2 is a cause rather than a consequence of colorectal carcinogenesis. The methylation of several gene promoters, such as CDKN2A, MGMT, MLH1 and vimentin, serves as a biomarker for early cancer detection using stool samples and as a tool for monitoring patients with CRCs [48] , [49] . The frequent methylation of RSPO2 in primary tumours, but not in the matched mucosa, makes RSPO2 a promising biomarker for the early detection of CRCs. In conclusion, we have shown that RSPO2 has important roles in CRC tumorigenesis. In CRC cells with a high level of LGR5 expression following RSPO2 treatment, RSPO2 interacts with LGR5 to stabilize membrane-associated ZNRF3 and thus suppresses Wnt/β-catenin signaling and tumour cell growth. Our studies have revealed a novel RSPO2-induced LGR5-dependent Wnt signaling-negative feedback mechanism that exerts a net growth-suppressive rather than growth-promoting effect on CRC cells. This finding indicates that in most human CRCs, RSPO2 functions as a Wnt signaling antagonist and as a tumour suppressor; therefore, it may represent a valuable molecular target for the development of therapies for CRCs. Tissue samples and cell lines Fresh primary colorectal tumours and matched adjacent normal mucosa with appropriate Institutional Review Board approval and patient-informed consent were obtained from the First Affiliated Hospital of Wenzhou Medical University. HEK293, LS174T, DLD1, HT29, HCT116 and other CRC cell lines were obtained from the American Type Culture Collection. Routine cell cultures were maintained in medium supplemented with 10% fetal bovine serum (FBS) and 1% penicillin/streptomycin and incubated in a 5% CO 2 atmosphere at 37 °C. Experiments with exogenous RSPO2 protein stimulation, RSPO2 overexpression or si-RSPO2 knockdown were performed in medium containing 5% FBS. Human LRP6 (#3395S), phospho-LRP6 (Ser1490) (#2568S), β-catenin (#9587S), c-Myc (#5605S), CD44 (#3570S) and β-actin (#4970S) antibodies were purchased from Cell Signaling Technology. Wnt3a and recombinant human RSPO1, 2, 3 and 4 proteins were obtained from R&D Systems. ZNRF3 (sc-86958), Cyclin D1 (sc-20044) and RSPO2 (sc-74883) antibodies were purchased from Santa Cruz Biotechnology. LGR5 (AP22745d) and IR-β (ab69508) antibodies were purchased from Abgent and Abcam, respectively. Plasmids N-terminal-tagged full-length human LGR4, LGR5 and LRP6 plasmids were gifts from Qingyun Liu (University of Texas-Houston Health Science Center, Houston, TX, USA). The TopFlash, FopFlash and pRL-TK plasmids were obtained from Promega. The full-length human RSPO2 cDNA was amplified from HEK293 cells using the One-Step RT-PCR System kit (Invitrogen), subcloned into pcDNA3.1 (Invitrogen) and verified by DNA sequencing. Quantitative real-time PCR (qRT–PCR) Total RNA was isolated from CRC cell lines and tumour samples using TRIZOL reagent (Invitrogen). A total of 2 μg of total RNA was reverse-transcribed to cDNA with MLV-reverse transcriptase (Invitrogen), and each cDNA sample was analysed in triplicate on an ABI 7300 Real-Time Detection system (Applied Biosystems) using SYBR Green (Tiangen, China) according to the manufacturer’s protocol. Endogenous housekeeping genes ( β-actin or GAPDH ) were used as internal standards. Cycle conditions were as follows: 95 °C for 2 min followed by 40 cycles of 95 °C for 15 s, 60 °C for 30 s and 68 °C for 30 s. Primer sequences are listed in Supplementary Table 1 . The relative quantification of the mRNA was calculated using the comparative threshold cycle ( C t ) method [50] . When necessary, we converted ΔΔ C t to a fold change of expression using the formula 2 −ΔΔ C t . Transient and stable transfection Transfections were performed using Lipofectamine 2000 reagent (Invitrogen) according to the manufacturer’s instructions. pEGFP-N1 (Clontech) was co-transfected to assess transfection efficiency. To obtain stable transfectants, the transfected cells were grown in medium with G418, and resistant clones were confirmed using western blotting. RSPO2 copy number determination The gene copy number of RSPO2 within the genome was determined with the TaqMan copy number assay (Applied Biosystems) according to the manufacturer’s protocol. Genomic DNA isolated from the tissue samples was used as a template. The probed RSPO2 primer (Hs02769963_cn) was run as a triplex TaqMan real-time PCR with RNase P as the reference gene, and HCT116 cells containing two copies of RSPO2 were used as a calibrator. Real-time PCR data were analysed by the threshold cycle ( C t ) method to calculate relative changes in the copy number of RSPO2. Bisulphite sequencing PCR (BSP) and methylation-specific PCR Genomic DNA was isolated with a Cell/Tissue DNA Extraction kit (BioTeke, China), and the bisulphite modification of genomic DNA was performed using an EZ DNA Methylation-gold kit (Zymo Research Corporation). CpG island analysis and primer design for BSP and MSP were performed with the Methyl Primer Express v1.0 software and the primers are listed in online Supplementary Table 1 . The BSP products were sequenced and analysed with the QUMA program ( http://quma.cdb.riken.jp/ ). The MSP products were analysed using agarose gel electrophoresis. β-Catenin reporter assay An RSPO2 expression plasmid (0–100 ng) and a β-catenin reporter pTopFlash (100 ng) were co-transfected into cells cultured in 24-well plates using Lipofectamine 2000 reagent (Invitrogen). A total of 2 ng of pRL-TK (Renilla luciferase) was co-transfected as an internal control. Forty-eight hours after transfection, the luciferase reporter assay was performed using the Dual-luciferase Reporter Assay System (Promega). To control for transfection efficiency, firefly luciferase levels were normalized to Renilla luciferase levels to generate a measure of relative luciferase units. An Envision Luminometer (Perkin-Elmer) was used to detect luminescence. Cells stably expressing the TopFlash reporter gene were used to examine the effect of exogenous RSPO2 protein, and luciferase activity was measured 12 h after RSPO2 protein addition. For the LGR5–RSPO2 co-transfection reporter assay, 100 ng of RSPO2 expression plasmid was used. Experimental data are presented as the means±s.d. of three independent wells. Small interfering RNA siRNA duplexes (SMARTpool PLUS) were purchased from Dharmacon Research. The target sequences of RSPO2 (si-RSPO2), LGR4 (si-LGR4) and LGR5 (si-LGR5) and the non-targeting sequences are listed in Supplementary Table 2 . Cells grown to a confluence of 50–70% were transfected with siRNA using Transfection Reagent (Dharmacon Research) and plated again for further experiments. The knockdown efficiency was determined using qRT–PCR or western blotting. As the RSPO2 protein levels were undetectable in LS174T and DLD1 parent cell lines, the siRNA knockdown experiment was performed on their stable RSPO2-transfected clones. MTT assay and clonogenic assay Cell viability was determined with the MTT (Sigma) assay as described previously [51] . For the clonogenic assay, cells were seeded in a 12-well plate and transfected with an equal amount of RSPO2 expression vector or the control pcDNA3.1 vector. Cells were selected for 2 weeks in a medium containing 5% FBS and 1,000 μg ml −1 G418. The surviving colonies were stained with 0.1% crystal violet, and colonies with more than 50 cells were counted. The clonogenic assay with stable RSPO2-overexpressing cells was performed in six-well plates using 500–1,000 cells that were seeded and maintained in medium with 5% FBS for 10 days. Xenograft Six-week-old male athymic nude mice (nu/nu) were purchased from Vital River Experimental Animal Center (Beijing, China) and maintained under pathogen-free conditions. The vector control and stable RSPO2-overexpressing LS174T, HCT116 or DLD1 cells were harvested and resuspended in PBS. A total of 5 × 10 6 cells in 100 μl PBS was subcutaneously injected in the rear flank of the mice. Tumour volumes were measured with a caliper and calculated as v = A × B 2 × 0.5326 ( A =long axis, B =short axis). At the end of the experiments, mice were killed, and the tumours were harvested and weighed. All animals were maintained and used in accordance with the guidelines of the Institutional Animal Care and Use Committee of Wenzhou Medical University. Western blotting Protein levels were determined by western blotting as described previously [52] . Briefly, cells were washed and lysed in lysis buffer supplemented with Protease/Phosphatase Inhibitor Cocktail (Cell Signaling Technology). After incubation on ice for 20 min, the lysate was centrifuged at 12,000 r.p.m. for 20 min at 4 °C, and the supernatant was collected. To prepare cytosolic (non-membrane bound) β-catenin, cell lysates were treated with ConA-sepharose beads (Amersham) for 4 h and then centrifuged to remove the cadherin-bound β-catenin. Cell-surface proteins were isolated by whole-cell biotinylation and avidin agarose pull-down using the Cell Surface Protein Isolation Kit (Pierce) according to the manufacturer’s instructions. Proteins were separated using SDS–polyacrylamide gel electrophoresis and transferred to polyvinylidene difluoride membranes (Bio-Rad). After blocking in 5% milk in TBST (0.1% Tween-20), the membranes were incubated with primary antibodies (1:500–1,000) followed by horseradish peroxidase (HRP)-conjugated secondary antibodies. Protein bands were visualized with the Immun-Star HRP Chemiluminescence kit (Bio-Rad). The full blots of the most important western blots are shown in Supplementary Fig. 15 . Immunofluorescence imaging The immunofluorescence analysis was performed as described previously [51] . Briefly, cells were seeded on coverslips for 40 h and then stimulated without (control) or with the RSPO2 protein (40 ng ml −1 ) for either 5 h (β-catenin detection) or 80 min and 4 h (LGR5 detection). After gentle washes with PBS, the cells were fixed with 4% formaldehyde and permeabilized with 0.5% Triton X-100 in PBS. Cells were subsequently blocked with 2% bovine serum albumin in PBS-0.1% Triton X-100 followed by incubation with primary antibody (diluted 1:100) at 4 °C overnight. After three washes with PBS-0.1% Triton X-100, samples were incubated with fluorescent-labeled secondary antibodies (diluted 1:1,000). Coverslips were mounted on glass slides in the presence of 4',6-diamidino-2-phenylindole for nuclear staining, and cell images were recorded using a ZEISS confocal microscope. Immunohistochemistry Colorectal tumours and their paired normal tissues were fixed in 10% formalin and embedded in paraffin blocks. Four-micrometre-thick consecutive sections were cut and mounted on glass slides. After deparaffinization, tissue sections were antigen-retrieved, washed and treated with peroxidase block (Santa Cruz Biotechnology). Then, sections were blocked with normal donkey serum and incubated with anti-RSPO2 antibody (Santa Cruz Biotechnology, diluted 1:100). After washing twice with PBS, the sections were incubated with biotinylated donkey-anti-goat secondary antibody and then with a horseradish peroxidase-streptavidin reagent (ImmunoCruz system, Santa Cruz Biotechnology). Colour was developed using a diaminobenzidine substrate. All sections were counterstained with diluted haematoxylin. A section incubated with normal goat serum without the RSPO2 antibody was used as a negative control. Sanger sequencing For RSPO2 gene fusion validation, we designed primers for PCR that generated an amplicon of 287 bp that contained the EIF3E promoter and the region of RSPO2 exon 2. The region in both tumours and matched mucosa was amplified using RT–PCR and then Sanger-sequenced. To investigate mutations in the LGR5 and RSPO2 promoters, a 1,129-bp promoter region of LGR5 and a 1,350-bp region of the RSPO2 promoter were amplified and sequenced. The primers used are listed in Supplementary Table 1 . Statistical analysis The data represent the mean±s.d. unless otherwise indicated. Statistical comparisons were performed using Student’s t -test. Significance was considered as P <0.05. The correlation between RSPO2 and LGR5 expression was evaluated by calculating the Spearman’s rank correlation coefficient using Statistical Package for the Social Sciences (SPSS) version 17.0. How to cite this article: Wu, C. et al . RSPO2–LGR5 signaling has tumour-suppressive activity in colorectal cancer. Nat. Commun. 5:3149 doi: 10.1038/ncomms4149 (2014). Accession codes: The RNAseq data have been deposited in the NCBI sequence read archive under accession code SRR1045067 .